Deterministic arbitrary switching of polarization in a ferroelectric thin film Ferroelectrics have been used as memory storage devices, with an upper bound on the total possible memory levels generally dictated by the number of degenerate states allowed by the symmetry of the ferroelectric phase. Here, we introduce a new concept for storage wherein the polarization can be rotated arbitrarily, effectively decoupling it from the crystallographic symmetry of the ferroelectric phase on the mesoscale. By using a Bi 5 Ti 3 FeO 15 -CoFe 2 O 4 film and via Band-Excitation Piezoresponse Force Microscopy, we show the ability to arbitrarily rotate polarization, create a spectrum of switched states, and suggest the reason for polarization rotation is an abundance of sub-50 nm nanodomains. Transmission electron microscopy-based strain mapping confirms significant local strain undulations imparted on the matrix by the CoFe 2 O 4 inclusions, which causes significant local disorder. These experiments point to controlled tuning of polarization rotation in a standard ferroelectric, and hence the potential to greatly extend the attainable densities for ferroelectric memories. Material properties in crystals are often determined by small perturbations of atoms from more symmetric lattice positions, with common examples including Jahn–Teller distortions in manganites [1] , octahedral cage rotations in perovskites [2] and cation displacements in ferroelectrics [3] . On the basis of the symmetry of the newly formed phase, the distortions may occur along one of several (that is, equivalent or energetically degenerate) directions, leading to material functionality if the population of such states can be effectively controlled. In a uniaxial ferroelectric perovskite, the central metal cation is displaced with respect to the surrounding octahedral oxygen anion cage, leading to the formation of a dipole moment and two possible polarization orientations, forming the basis of a bi-stable memory architecture that can be reversed through application of an electric field [4] . Early experiments with Piezoresponse Force Microscopy (PFM) on ferroelectric thin films of Pb(Zr x ,Ti 1− x )O 3 (PZT) by Tybell et al . [5] showed that, with an atomic force microscopy (AFM) tip, it is possible to write stable circular domains with radius as small as 20 nm, leading to theoretical densities on the order of ~Gbit cm −2 . However, in a planar capacitor setup, such a small radius would not be feasible, and other methods to increase density have been suggested. Lee et al . [6] proposed a multi-level memory storage system based on intermediate states between two polarization states −P s and +P s , modulated by limiting the current during the polarization switching process. Such a procedure should allow up ~10 × increase in density over current storage methods, and has the advantage of easy integration with existing architectures. More recently, a ‘ferroelectric memristor’ was demonstrated that showed a continuous spectrum of states, from −P s to +P s , and reading occurring through resistance changes through the metal/ferroelectric/metal device [7] . Another method that has been employed is to change from a uniaxial to a multiaxial system, such as rhombohedral BiFeO 3 , first demonstrated by Balke et al . [8] , or to a system with even more variants, such as monoclinic mixed-phase BiFeO 3, which has been shown by several groups [9] , [10] , [11] . In these cases, deterministic switching by means of an AFM probe motion has been shown, which has produced up to 16 distinct states [9] . In each of the above, the direction of switching is necessarily coupled to the long-range order parameter. On the other hand, one unexplored possibility is that of decoupling the polarization variants from the symmetry of the bulk (parent) material. That is, if the polarization vector can be arbitrarily rotated in space, theoretical densities could be increased by up to two orders of magnitude over current uniaxial ferroelectric setups. The existence of continuous polarization rotation in standard ferroelectrics was itself only confirmed recently by Jia et al . [12] through transmission electron microscopy studies, wherein flux-closure dipole structures were found in thin films of PZT, although they were known to exist for several decades through spectroscopic studies on relaxor ferroelectrics (‘relaxors’) such as Pb(Mg 1/3 Nb 2/3 )O 3 (ref. 13 ). Here, though the crystal structure is cubic, it is argued that due to charge disorder, there exist polar nanoregions that rotate and align with applied fields, resulting in large electromechanical response, but the structure lacks any long-range ordering. Since then, polarization rotation in standard ferroelectrics has been confirmed through several other transmission electron microscopy (TEM)-based studies [14] , [15] including across c/a ferroelastic domain boundaries in PZT thin films [16] . Energetically, polarization rotation of an individual dipole is necessarily costly, unless coupled to a larger flux-closure-like structure to minimize depolarization fields, and is therefore generally expected in situations where charge screening is limited. Alternatively, polarization rotation would be expected in situations where there is significant local disorder, whether it be compositional [17] , charge, or arise from strain effects, as the local crystallography could heavily deviate from the bulk in such instances and be accommodating to such lattice distortions, or when domain wall energies approach extremely small values, as in morphotropic phase boundary (MPB) ferroelectrics [18] , [19] , [20] . Indeed, polarization rotations are a crucial aspect of theories surrounding MPB ferroics and relaxors, that strive to explain the extremely large electromechanical responses found in these systems. These include those supporting low-symmetry monoclinic bridging phases [21] , thus allowing rotation through, for example, (110) plane, and others proposing an adaptive phase [18] structure with nanoscale texture, which due to vanishingly small polarization anisotropy, becomes decoupled and unstable against rotation. One of the important aspects of such behaviour should be polarization rotation in mesoscopic volumes, for example, comparable to signal formation region in X-rays, but evidence at these length scales is scant. Here, we show the possibility to rotate polarization on the mesoscale at any in-plane angle by using a moving, biased AFM tip, create a spectrum of switched states and effectively decouple the polarization from the symmetry of the parent phase at the mesoscopic scale without breaking ferroelectric order through Band-Excitation Piezoresponse Force Microscopy (BE-PFM) [22] , [23] . Our material of interest is the recently reported Bi 5 Ti 3 FeO 15 -CoFe 2 O 4 (BTFO–CFO) epitaxial multiferroic nanocomposite [24] , where the CFO nanopillars impart compressive stress to the BTFO matrix, inducing a ferroelectric phase transition, and inducing significant disorder. High-resolution BE-PFM scans, in combination with TEM-based strain mapping, reveals sub-50 nm size nanodomains which appear key in facilitating the mesoscopic polarization rotation in this material system. Lateral band-excitation PFM experiments The system studied is a 50 nm composite film of BTFO–CFO, the details of which have been published elsewhere [24] . In this film, CFO nanopillars inclusions impart a compressive stress on the ferroelectric BTFO film, inducing a phase transition to a new ferroelectric phase with a very weak out-of-plane component and a larger in-plane polarization [24] . The AFM topography of the film can be seen in Fig. 1a , along with a schematic of the writing process. The surface topography is not flat, due to the CFO inclusions, and can be expected to result in highly inhomogeneous local strain distributions as will be discussed later. As the tip is moved from one location to another, the symmetry of the field applied that converges at the tip (in the case of a negative bias) is broken, leading to a net E-field vector, plotted as a red arrow (‘Trailing Field’). By manipulating the angle at which the tip scans, it is then possible to align the polarization of the BTFO layer underneath the tip to this trailing field direction. An example of this is shown in the mixed lateral PFM image in Fig. 1b , where the tip was held at −12 V and scanned upwards for the first half of the scan, and then downwards for the second half (indicated by the red arrows). After the writing step, the lateral BE-PFM image was captured (the orientation of the cantilever during the measurements is indicated on the figure). BE-PFM allows decoupling of topographical cross-talk that is inherent in PFM measurements taken near the contact resonance frequency, and thus allows quantitative signal extraction [22] , [25] . Note that white points are points where the signal was too weak, and are excluded from analysis. Examples of points from the two written rectangles in Fig. 1b are shown in the amplitude and phase plots in Fig. 1c,d , respectively. These plots show the datapoints captured (filled circles) as a function of frequency, as well as their corresponding simple harmonic oscillator fits (solid lines), that are used to determine the final amplitude and phase throughout this manuscript. Here, it is important to note that the different points plotted in Fig. 1c suggest there is some imprint in the film that causes one polarization direction (in this case, [−100]) to exhibit a higher contrast than the opposite ([100]) direction. This can be more clearly seen in the BE-amplitude histogram for the (lateral) poled orientations in Fig. 1e . The imprint is presumably caused by defects that are formed on cooling and annealing of the samples. Nonetheless, the phase plot in Fig. 1d shows a clear phase change of about 180°, and this experiment proves the possibility of lateral writing on this film. At this point, we note that the origin of the lateral BE-PFM signal is definitely field-induced piezoelectric strain, and not other possibilities, such as surface charging and related electrostatics coupling with lateral modes of the cantilever. This is confirmed by the extremely weak vertical BE-PFM response of poled areas of these films, whereas the corresponding lateral areas show high lateral BE-PFM response ( Supplementary Fig. 1 ). 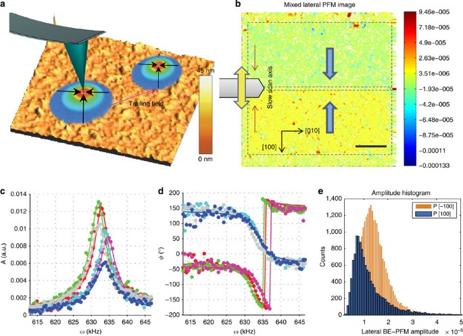Figure 1: Lateral BE-PFM of BFTO/CFO Composite Film. (a) Topography of sample and schematic of tip and ‘writing in wake’ effect. Two rectangles were then written with the tip biased at −12 V in this region, with the direction of the slow scan axis changed from [100] to [−100]. The results are shown inbMixed Lateral BE-PFM Image, and the location of the rectangles are indicated with the dashed boundaries. The red arrows indicate the direction of the slow scan axis used during the writing step. Scale bar, 1 μm. (c,d) Selected points from the BE-PFM image, showing the response (filled circles) at individual points as a function of frequency and the corresponding fit (simple harmonic oscillator/SHO, coloured lines), from which the amplitude and phase of the response at that point is determined and combined to produce the mixed BE-PFM image inb. The red, green and magenta points are from the upper switched portion, and the blue, cyan and grey curves are from the lower switched portion. The direction of the polarization vectors in the written rectangles are indicated by the blue arrows.eAmplitude Histogram of poled areas inb. Figure 1: Lateral BE-PFM of BFTO/CFO Composite Film. ( a ) Topography of sample and schematic of tip and ‘writing in wake’ effect. Two rectangles were then written with the tip biased at −12 V in this region, with the direction of the slow scan axis changed from [100] to [−100]. The results are shown in b Mixed Lateral BE-PFM Image, and the location of the rectangles are indicated with the dashed boundaries. The red arrows indicate the direction of the slow scan axis used during the writing step. Scale bar, 1 μm. ( c , d ) Selected points from the BE-PFM image, showing the response (filled circles) at individual points as a function of frequency and the corresponding fit (simple harmonic oscillator/SHO, coloured lines), from which the amplitude and phase of the response at that point is determined and combined to produce the mixed BE-PFM image in b . The red, green and magenta points are from the upper switched portion, and the blue, cyan and grey curves are from the lower switched portion. The direction of the polarization vectors in the written rectangles are indicated by the blue arrows. e Amplitude Histogram of poled areas in b . Full size image Next, to explore the dependence of the switching on the bias applied to the tip, a square was written with the bias varied progressively from −10 to −12 V as the tip was scanned downwards for the top half, and upwards for the lower half, as indicated in the BE-PFM amplitude and phase images in Fig. 2a,b . The region that was subjected to the bias is indicated by the black outlined region in Fig. 2a,b . Average line profiles for the BE-PFM amplitude and phase were computed for sections from the lower and upper halves, and are are shown in Fig. 2c and Fig. 2d , respectively. The error bars indicate 95% confidence intervals for the data. Note that these line profiles begin a few lines outside the black outlined square (starting in the unpoled region) to better aid comparison between the poled and unpoled areas. The profile indicates that there appears to be a transition between the poled and upoled areas, that is, a partially poled region appears, which is about 15 lines in width in both Fig. 2c,d , and the amplitude and phase appear to smoothly increase in this region (neglecting surface defects). Therefore, varying the bias applied to the tip allows a spectrum of switched states, similar to previous work [6] , [7] , [26] . 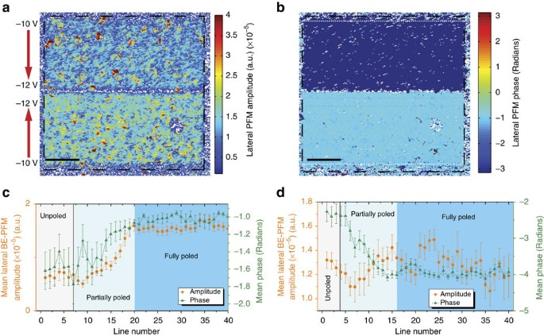Figure 2: Creating a spectrum of switched states. Progressive poling by negative tip bias, with the tip bias increased from −10 to −12 V with the tip scanning downwards (top half) and upwards (lower half) is shown in the lateral BE-PFM amplitude (a) and phase (b) images. The black outlined box indicates the edge of the area where the bias was applied to the tip. Black scale bars are 1.6 μm. At the upper and lower edges, this results in small areas that are partially poled, since these regions are exposed to a smaller effective lateral field component than the more interior regions. Line averages of the BE-amplitude and phase for the (c) lower half and (d) upper half of the images are graphed with the 95% confidence intervals. Note that these graphs begin just outside the black outlined regions(that is, start of poling), and cut off after 40 lines. The dotted line inbindicates, approximately, the boundary between the partially poled and fully poled regions. Figure 2: Creating a spectrum of switched states. Progressive poling by negative tip bias, with the tip bias increased from −10 to −12 V with the tip scanning downwards (top half) and upwards (lower half) is shown in the lateral BE-PFM amplitude ( a ) and phase ( b ) images. The black outlined box indicates the edge of the area where the bias was applied to the tip. Black scale bars are 1.6 μm. At the upper and lower edges, this results in small areas that are partially poled, since these regions are exposed to a smaller effective lateral field component than the more interior regions. Line averages of the BE-amplitude and phase for the ( c ) lower half and ( d ) upper half of the images are graphed with the 95% confidence intervals. Note that these graphs begin just outside the black outlined regions(that is, start of poling), and cut off after 40 lines. The dotted line in b indicates, approximately, the boundary between the partially poled and fully poled regions. Full size image Evidence for nanodomains The ability to create a spectrum of switched states in this material can be expected for any ferroelectric that consists of nanodomains. Due to disorder, each nanodomain will have a different coercive field, resulting in partial switching of poled areas consisting of large numbers of nanodomains for some intermediate range of applied fields. To ascertain more information about local disorder, we employed a combination of high-resolution BE-PFM and TEM-based strain mapping. The topography of a 500 × 500 nm area of a poled area of the sample is shown in Fig. 3a , and the lateral BE-PFM amplitude image is shown in Fig. 3b . Numerous areas of low or minimal response (dark–light blue colours) can be seen in the image, which are characteristic of the CFO nanopillars (as these are not ferroelectric). However, the BTFO film shows an abundance of ~50 nm nanodomains, which show a range of amplitudes. The driving force for the nanodomains appears to be the inclusion of the CFO nanopillars, which exerts a compressive stress on the BTFO film. Indeed, the pressure is extremely large, on the order of ~1–3 GPa, which transforms the non-ferroelectric BTFO film into a ferroelectric film with weak out-of-plane polarization and much stronger in-plane polarization [24] . To observe the effect of the CFO nanopillars on the lattice structure, we undertook strain mapping through geometric phase analysis, [27] as shown in Fig. 3c . In this image, the film is imaged along the (010) zone axis. The coloured scale bar shows the lattice parameter changes relative to the a-axis parameter of CFO inclusions (0.418 nm in pseudocubic notation). The mismatch strain between BTFO film and CFO inslusions is calculated to be 8.15% in-plane and 1.93% the out-of-plane. This is large enough to create misfit dislocations along the tubular interface. Wave-like patterns can be seen to propagate through the BTFO film as a result of the CFO inclusion, which suggest that the stress distribution is extremely inhomogeneous. This disorder likely lies at the heart of the nanodomain structure, and importantly could also allow the polarization to rotate arbitrarily without preference to a bulk crystal symmtery axis. Here, we posit the following scenario for deterministic arbitrary writing of polarization on the mesoscale: applying a negative tip bias and scanning, for example, downwards, as shown in the schematic in Fig. 3d , produces a net electric in-plane field aligned along the slow scan axis, but since the cantilever is scanning back and forth along the fast scan axis (FSA), domains are constantly being rewritten. We may then expect that the local polarization will attempt to align along the net E direction, but be affected by the fluctuations due to local disorder and the last field the domain experienced. Note that in this scenario, the local dipoles may still remain coupled to the crystallographic symmetry (which may be monoclinic [24] ). However, on the mesoscale, the result is a collection of nanodomains in the BTFO that are switched with a net polarization P that is along E, but with local departures, as indicated in the figure. Thus, the assortment of nanodomains behaves as a domain with rotatable, arbitrary polarization vector on the mesoscale. 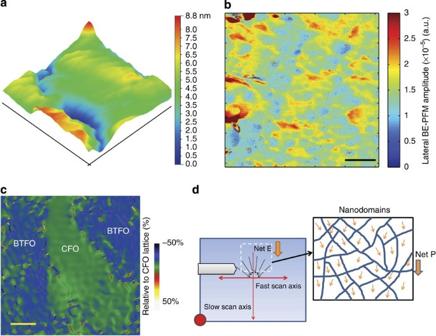Figure 3: High-resolution BE-PFM and TEM studies. Topography (0.5 × 0.5 μm) (a) and Lateral BE-PFM amplitude image (b) after poling with −11 V. Many small domains smaller than 50 nm in size can be seen in this image. The scale bar (black line) is 100 nm in length. (c) Strain mapping confirms the strain distribution is highly inhomogeneous around the CFO pillars, as indicated by the blue ripples that permeate the BFTO matrix. Such inhomogeneous stresses can cause the formation of nanodomains, due to the local disorder (analogous to nanodomains in MPB ferroelectrics, for example). Yellow scale bar, 10 nm. (d) Schematic of the lateral writing by the tip. As the negatively biased tip scans downwards, the polarization in the nanodomains align to the trailing field, which (vector) sum to the slow scan axis (SSA). Figure 3: High-resolution BE-PFM and TEM studies. Topography (0.5 × 0.5 μm) ( a ) and Lateral BE-PFM amplitude image ( b ) after poling with −11 V. Many small domains smaller than 50 nm in size can be seen in this image. The scale bar (black line) is 100 nm in length. ( c ) Strain mapping confirms the strain distribution is highly inhomogeneous around the CFO pillars, as indicated by the blue ripples that permeate the BFTO matrix. Such inhomogeneous stresses can cause the formation of nanodomains, due to the local disorder (analogous to nanodomains in MPB ferroelectrics, for example). Yellow scale bar, 10 nm. ( d ) Schematic of the lateral writing by the tip. As the negatively biased tip scans downwards, the polarization in the nanodomains align to the trailing field, which (vector) sum to the slow scan axis (SSA). Full size image Arbitrary writing To test whether the polarization vector can indeed be rotated arbitrarily in this manner, nine squares were written with the tip scanning upwards, with the tip biased at −12 V to ensure complete switching, with the scan angle varied from 10 to 90°. As the tip is engaged in line-by-line scanning, each line being scanned is parallel to the FSA, while the vector from one scanned line to the next (or overall direction of the scan) defines the slow scan axis (SSA), and is perpendicular to the FSA. The scan angle refers to the angle that the FSA makes with the [0–10/010] axes, as indicated in Fig. 4a during the writing step. In effect, the trailing field becomes aligned along the SSA in these writing experiments, assuming a negative tip bias and upward tip motion. After the squares were written, a lateral BE-PFM image was taken (with a scan angle of 0°), which is shown in the amplitude and phase images in Fig. 4a,b . In the colour scheme used, blue colours for phase indicate in-plane polarization orientations along [−100], while red colours indicate in-plane polarization orientations along [100]. For the BTFO film, though the symmetry is monoclinic [24] , the variants should be very closely aligned along the <100> axes, corresponding to scan angles of 0 and 90° for this setup. Applying a field at 30–60° to <100> should result in frustration and partial switching, but it does not appear to be the case, because the measured phase for these write angles indicates little change, as can be seen in the plot of amplitude versus phase for the nine written squares, in Fig. 4c . This graph indicates that the average phase for the written squares is remarkably stable up to ~70°, after which it changes, but the amplitude appears to obey the expected cosine dependence through the measured theta range. For non-arbitrary polarization rotation, amplitude would still obey cosine theta dependence, but this would arise from switched fractions decreasing, as there is a decreasing fraction of domains with coercive fields below the applied field, that is, the average phase should also obey a cosine dependence, which is not seen in our case. At very high angles, there appears to be an increasing fraction of domains with (very weak) in-plane polarization components along [100], as indicated by the red regions in the phase image in Fig. 4b . This is probably caused by polarization vectors that are actually aligned along [010], but will produce a small lateral signal due to imperfect cantilever alignment. We reason that this switching along [010] at high angles is due to the fact that the field application by tip is not perfectly unidirectional, and may be exacerbated by film imprint effects. 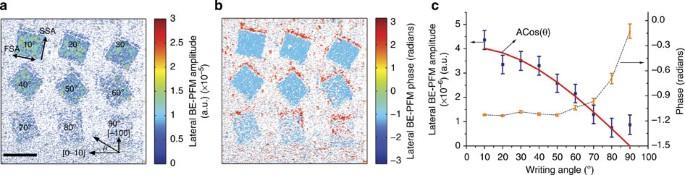Figure 4: Writing as a function of tip scan angle. Writing was carried out in 2 × 2 μm boxes with the tip scanning upwards and biased at −12 V, but with the scan angle varied in 10° increments from 10 to 90°, as shown in the Lateral BE-PFM amplitude (a) and Phase (b) images. Scale bar, 3 μm. The scan angle refers to the angle subtended by the cantilever scanning along the FSA and the [0–10/010] axis as indicated in the figure. With the tip/cantilever scanning upwards with a negative bias, the trailing field (and hence polarization) becomes aligned along the SSA. The average amplitude and phase from the written squares is plotted in (c). The amplitude (squares) of the signal decays as a cosine of the theta (where theta is the write angle, a fit is shown as a solid red line); however, the phase (triangles, indicating switched fraction) remains remarkably constant until about 70°, which would be consistent with arbitrary polarization switching. For angles greater than 70°, the phase changes, and the image indicates that some regions are switching (probably along [010]). Figure 4: Writing as a function of tip scan angle. Writing was carried out in 2 × 2 μm boxes with the tip scanning upwards and biased at −12 V, but with the scan angle varied in 10° increments from 10 to 90°, as shown in the Lateral BE-PFM amplitude ( a ) and Phase ( b ) images. Scale bar, 3 μm. The scan angle refers to the angle subtended by the cantilever scanning along the FSA and the [0–10/010] axis as indicated in the figure. With the tip/cantilever scanning upwards with a negative bias, the trailing field (and hence polarization) becomes aligned along the SSA. The average amplitude and phase from the written squares is plotted in ( c ). The amplitude (squares) of the signal decays as a cosine of the theta (where theta is the write angle, a fit is shown as a solid red line); however, the phase (triangles, indicating switched fraction) remains remarkably constant until about 70°, which would be consistent with arbitrary polarization switching. For angles greater than 70°, the phase changes, and the image indicates that some regions are switching (probably along [010]). Full size image We note here that there are two relevant variables to determine the final polarization orientation of the written domains: the scanning angle of the cantilever, and the relative orientation of the sample. In the previous case, the sample orientation was kept constant, and the scanning angle was varied incrementally. Next, we test the second variation where the scanning angle is kept fixed at 0° and instead the sample is rotated (by eye), in 15° increments from 0 to 90°. In total, seven squares were written with the tip scanning upwards with tip bias of −12 V. After the writing, three BE-PFM scans were taken with the sample rotated at 0, 45 and 90° to [100] check the amplitude and phase of the written squares. As a guide, the orientation of the sample with respect to the cantilever is shown by the cartoon schematics in each image. To confirm that each square was fully switched, single-frequency PFM images were captured after each writing step ( Supplementary Fig. 2 ). The BE-PFM amplitude images from this experiment are indicated in Fig. 5a–c for the three different angles; phase images are provided ( Supplementary Fig. 3 ). Note again that in each BE-PFM image shown, the scan angle during image capture was kept to 0°. The amplitudes of the written squares were then calculated for the three different orientations from the BE-PFM amplitude images, with a subtraction of the background to ensure that squares written at 90° and read at 0° would average to zero amplitude (in the ideal case). The resulting plot is shown in Fig. 5d , with the trends for the 0 and 90° scans showing the expected cosine and sine dependence, and a cross-over at 45°. 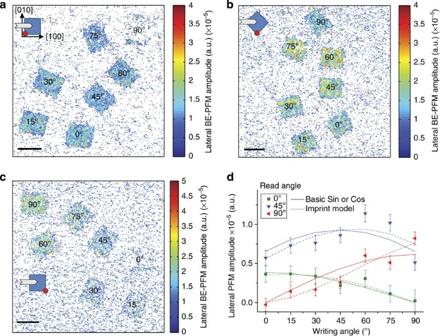Figure 5: Writing with sample rotation. Writing was carried out at an optimal angle (0° scan angle), but with the sample in seven different orientations, and the PFM images were recorded with the sample in three different orientations after the writing. The orientation of the sample during the imaging steps is indicated with the cartoon schematics. Single-frequency PFM after each writing step confirms full writing of each square (Supplementary Fig. 2). Lateral BE-PFM scans with the sample oriented at (a) 0°, (b) 45° and (c) 90° to [100] are shown. All scale bars are 2 μm The average amplitude in each of the written squares, calculated from the amplitude images, is plotted ind. Note that the background has been subtracted from each mean amplitude. The graph shows that for the different written boxes, the amplitude follows the expected dependency based on arbitrary writing of polarization. The 45° scan shows that boxes written with the sample at somewhat higher angle offsets have larger amplitudes, but this is due to some imprint in the material, and can also be seen inFig. 1. The cosine fits are shown as solid lines, and the slightly more complex function taking imprint into consideration is plotted as a dashed line. Mathematically, the lateral BE-PFM amplitude L of the nth square, which was written with writing angle θ n for a given sample orientation α , is given by: Figure 5: Writing with sample rotation. Writing was carried out at an optimal angle (0° scan angle), but with the sample in seven different orientations, and the PFM images were recorded with the sample in three different orientations after the writing. The orientation of the sample during the imaging steps is indicated with the cartoon schematics. Single-frequency PFM after each writing step confirms full writing of each square ( Supplementary Fig. 2 ). Lateral BE-PFM scans with the sample oriented at ( a ) 0°, ( b ) 45° and ( c ) 90° to [100] are shown. All scale bars are 2 μm The average amplitude in each of the written squares, calculated from the amplitude images, is plotted in d . Note that the background has been subtracted from each mean amplitude. The graph shows that for the different written boxes, the amplitude follows the expected dependency based on arbitrary writing of polarization. The 45° scan shows that boxes written with the sample at somewhat higher angle offsets have larger amplitudes, but this is due to some imprint in the material, and can also be seen in Fig. 1 . The cosine fits are shown as solid lines, and the slightly more complex function taking imprint into consideration is plotted as a dashed line. Full size image where θ n ={15,30,45,60,75,90°} and α ={0,45,90°}. Since single-frequency PFM confirms that all of these squares have been fully poled, the reduction in amplitudes of the written squares in the same BE-PFM image is clear evidence of arbitrary polarization writing in this film (for more detailed discussion, please see Supplementary Discussion ). For the 45° case, one would expect a peak to appear at 45° and a reduction on either side, but here there appears to be a peak closer to 60°. We reason that this is due to the imprint in the film, which can be also seen in Fig. 1b,e , which tends to result in higher amplitudes for squares written at higher angles. This imprint may be semi-quantified by a simple modification to equation (1), that is, if we now assume that A n = A 0 + θ n k , varying linearly by some parameter k . Fitting using this relationship is indicated by the dashed lines in Fig. 5d . Surprisingly, despite the simplicity of this model, there is some better agreement with the obtained data using this imprint model. Essentially, poor adherence to the cosine relationship may be expected when kθ n becomes comparable in magnitude to A 0 , since then differences in amplitudes would become dominated by the A n term rather than the cosine term. The effect of this would be to require very large separation angles such that the cosine term dominates again to exacerbate differences between squares written at different angles. We note here that a pure film of BTFO, without any CFO inclusions, does not show any nanodomains, and could not even be poled easily ( Supplementary Figs 4 and 5 ), suggesting that these nanodomains are a necessary prerequisite for arbitrary polarization writing. Further, while there is a long distance from these experimental observations to a fully integrated practical device, these results suggest the potential for ferroelectric memory storage systems with lateral planar electrode geometries [28] , [29] , [30] , which can greatly increase the possible density of storage with less leakage issues. Vertical memory architectures can suffer with depolarization field effects, which competes with and can destroy the ferroelectricity in ultrathin geometries [31] , but these problems are considerable reduced in the lateral writing scheme, as there is no polarization disontinuity at the film’s surface (polarization is parallel to the surface for all lateral directions). Future challenges will lie in developing suitable read mechanisms. On a fundamental level, the existence of continuous polarization rotation in standard ferroelectrics was itself controversial until very recently; here, we illustrate a novel system where it not only exists on the mesoscale, but can be manipulated by external electric fields. That is, here we have direct evidence of mesoscale deterministic polariation rotations in ferroelectric thin film, proving that the polarization rotations that are the cornerstone of theories of high electromcehcanical response in the realxor ferroelectrics and MPB ferroelectrics (whether through adaptive phases, or through bridging phases) can indeed take place, at least in this system. Finally, we note that the retention of the written domains is considerable, probably due to the intrinsic disorder-induced pinning: scans of the written squares show only 30% change in amplitude over 24 h ( Supplementary Fig. 6 ). Film preparation The sample films were prepared by pulsed laser deposition. The BTFO–CFO composite (CFO: ~30 vol %) film (~50 nm in thickness) was grown by alternate depositon of Bi 4 Ti 3 O 12 and CoFe 2 O 4 targets in 500 mTorr O 2 at 690 °C the details of which have been published elsewhere [24] . The BTFO pure film (~40 nm in thickness) was grown from a pure BTFO target in 50 mTorr O 2 at 600 °C. PFM experiments Arbitary writing experiments were performed on a commercially available atomic force microscope (Asylum Research, Cypher Brand) in ambient conditions equipped with in-house band-excitation performed with National Instruments PXI-based electronics with Labview and Matlab-based scripts. Numerical analysis was performed with scripts written in Matlab v2013b. Error calculation Error bars in all graphs are the 95% confidence intervals, calculated by where μ is the mean, t is the Student’s t -distribution two-tailed probability, n is the number of observations (points in the dataset), and s is the s.d. of the dataset. How to cite this article: Vasudevan, R. K. et al . Deterministic arbitrary switching of polarization in a ferroelectric thin film. Nat. Commun. 5:4971 doi: 10.1038/ncomms5971 (2014).